A molecular pathway for CO2response inArabidopsisguard cells Increasing carbon dioxide (CO 2 ) levels in the atmosphere have caused global metabolic changes in diverse plant species. CO 2 is not only a carbon donor for photosynthesis but also an environmental signal that regulates stomatal movements and thereby controls plant–water relationships and carbon metabolism. However, the mechanism underlying CO 2 sensing in stomatal guard cells remains unclear. Here we report characterization of Arabidopsis RESISTANT TO HIGH CO 2 (RHC1), a MATE-type transporter that links elevated CO 2 concentration to repression of HT1, a protein kinase that negatively regulates CO 2 -induced stomatal closing. We also show that HT1 phosphorylates and inactivates OST1, a kinase which is essential for the activation of the SLAC1 anion channel and stomatal closing. Combining genetic, biochemical and electrophysiological evidence, we reconstituted the molecular relay from CO 2 to SLAC1 activation, thus establishing a core pathway for CO 2 signalling in plant guard cells. Stomatal pores are responsible for gas exchange between plants and the atmosphere, thereby controlling plant–water relationships and carbon metabolism. Stomatal opening/closing is thus considered as a main switch for carbon cycling in the ecosystem. Under normal conditions, stomata of most land plants close in response to high carbon dioxide (CO 2 ) concentrations and open at low CO 2 concentration. The continuing rise in atmospheric CO 2 concentration reduces stomatal apertures across diverse plant species and alters plant metabolism on a global scale [1] . However, the mechanism by which CO 2 controls stomatal movements remains unclear. Stomatal movement is regulated by the transport of inorganic ions and organic metabolites across guard cell membranes [2] , [3] , [4] , [5] , [6] . Elevated CO 2 concentration activates anion channels, resulting in depolarization of plasma membrane in guard cells, causing efflux of solutes and stomatal closure [7] , [8] , [9] , [10] . Earlier studies in Arabidopsis identified several mutants with defects in CO 2 -induced stomatal movements [11] , [12] , [13] , [14] , [15] , [16] , [17] , [18] , [19] . However, most of these mutants including abi1-1 , abi2-1 , gca2 , ost1 and slac1 were insensitive to both CO 2 and abscisic acid (ABA), representing components shared by both signalling pathways [5] , [20] . Activation of the slow (S-type) anion channels for anion efflux has been regarded as a critical step in stomatal closure [18] , [21] , [22] , [23] , [24] . SLAC1 (Slow Anion Channel-Associated 1) is a component of the S-type anion channel in Arabidopsis guard cells [14] , [15] . When expressed in Xenopus oocytes, SLAC1 forms a channel that is permeable to Cl − and NO 3 − , but not to HCO 3 − [23] , [24] . In addition to SLAC1, Arabidopsis guard cells also express SLAH3, a second S-type anion channel [25] , which is especially important for the extrusion of NO 3 − . In contrast to S-type channels, R-/QUAC-type anion channels may be essential for the efflux of organic acids such as malate, which can accumulate during stomatal opening and be released during closure [26] , [27] , [28] . A group of kinases such as OST1 (STOMATAL OPEN 1), CPKs (Ca 2+ -dependent protein kinases) and GHR1 (GUARD CELL HYDROGEN PEROXIDE-RESISTANT 1) can phosphorylate and activate the SLAC1 anion channel [23] , [24] , [29] , [30] , [31] , [32] . Such activation is often considered to be the key step for ABA-induced stomatal closure [21] , [22] , [23] , [24] . OST1 can also interact and activate R-type channel QUAC1 (ref. 33 ). Therefore, OST1 is a central transducer of ABA and CO 2 signal pathways in guard cells [6] , [18] . The HT1 (HIGH LEAF TEMPERATURE 1) [13] and carbonic anhydrase (CA) [17] are two components that appear to specifically function in the CO 2 -sensing pathway. The HT1 gene encodes a protein kinase that is expressed predominantly in guard cells and functions as a major negative regulator of CO 2 -induced stomatal closing. The ht1-1 and ht1-2 mutants exhibit constitutive high CO 2 response, closing their stomata under both low- and high-CO 2 conditions [13] . In contrast, Arabidopsis mutant plants disrupted in βCA1 and βCA4 ( ca1ca4 double-mutant) are strongly impaired in stomatal CO 2 responses, suggesting that CAs, unlike HT1, are positive regulators of CO 2 response. Interestingly, expression of a mammalian α-CA in guard cells of the ca1ca4 double-mutant restores stomatal CO 2 response, indicating that CA-mediated CO 2 conversion into bicarbonate is an initial step for transmission of the CO 2 signal [17] , [34] . A further study demonstrates that intracellular bicarbonate produced by CA activates the S-type anion channels in guard cells, leading to ionic efflux, thus triggering the closure of stomatal pores [18] . Consistent with this conclusion, in mammalian cells, CO 2 detection in olfactory receptor neurons also starts with CA catalysis of CO 2 into bicarbonate, followed by activation of the receptor-type guanylate cyclase GC-D [35] , [36] , [37] . While several components in the CO 2 response pathway have been identified using a genetic approach in Arabidopsis , the relationship of the identified components is unknown and some important components remain to be discovered. To further dissect the CO 2 signalling pathway, we combined candidate-gene analysis and a phenotypic screen of genetic mutants to identify proteins involved in high CO 2 response. We report here the identification of a MATE (MULTIDRUG AND TOXIC COMPOUND EXTRUSION)-like protein, RHC1 (RESISTANT TO HIGH CARBON DIOXIDE 1), as an essential component for CO 2 -induced stomatal closure. We further demonstrate that RHC1 serves as an upstream regulator of HT1 that in turn inhibits OST1, connecting the CO 2 -specific pathway to OST1–SLAC1 activation, a common step shared by the ABA and CO 2 responses. The rhc1 mutant is defective in stomatal response to CO 2 Although several proteins have been shown to function in CO 2 -regulated stomatal response, some critical components are still missing [5] , [6] , [18] . Because membrane transporters play an important role in modulating stomatal response to external signals [5] , [6] , [14] , [15] , [16] , [38] , [39] , [40] , we hypothesized that mutations in many of such transporters may affect stomatal responses to environmental signals including CO 2 concentration. We identified a large number of genes encoding potential solute transporters and collected T-DNA insertion mutants for these genes to compile a mutant library. We subjected this mutant library to a phenotypic screen in a high-CO 2 (700 p.p.m.) growth chamber. Under this condition, wild-type (WT) (Columbia, Col-0) plants showed stunted growth phenotype as compared with those grown under the ambient CO 2 conditions. A mutant line (SALK_123674), rhc1 , showed more rapid leaf expansion as compared with the WT plants under the 700 p.p.m. CO 2 condition ( Supplementary Fig. 1a ). Under standard growth conditions, the rhc1 mutant plants were indistinguishable from the WT ( Supplementary Fig. 1b ). The mutant harboured a single T-DNA insertion in the exon of the At4g22790 gene, encoding a member of the MATE family ( Supplementary Fig. 1c ) [41] , [42] . The RHC1 gene encodes a predicted protein of 491 amino acids with 12 predicted transmembrane helices and hydrophilic amino- and carboxy-terminal tails (36 and 34 amino acids, respectively) ( Supplementary Fig. 2 ). Using reverse transcription–PCR, we confirmed that there was no detectable RHC1 transcript in the homozygous rhc1 mutant plants ( Supplementary Fig. 1d ). A WT genomic copy of RHC1 complemented the mutant phenotype in stably transformed rhc1 ( Supplementary Fig. 1a,b,d ). Tissue expression profiles of the RHC1 gene were analysed in transgenic plants carrying the RHC1 promoter ::beta-glucuronidase ( GUS ) gene reporter. Histochemical GUS-activity analysis indicated that the RHC1 promoter is highly active in the guard cells. Lower levels of activity were also identified in other tissues including vasculature ( Fig. 1a–e ). Transient expression of a 35S::RHC1–GFP fusion construct in Arabidopsis thaliana protoplasts revealed that RHC1 is targeted to the plasma membrane, similar to the pattern of the green fluorescent protein (GFP) fusion of SLAC1 that is a plasma membrane-localized anion channel [14] , [15] ( Fig. 1f ; Supplementary Fig. 3 ). 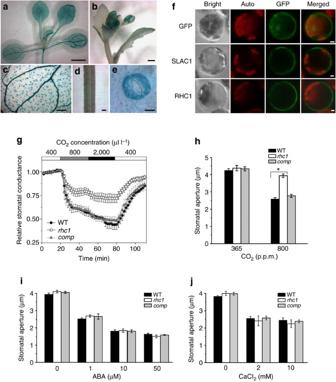Figure 1: Therhc1mutant plants are defective in stomatal responses to CO2. (a–e) Expression ofRHC1::GUSin leaves (a), flowers (b), vascular systems (c), stem (d) and guard cells (e). Scale bars, 500 μm (a,b), 100 μm (c,d), 5 μm (e). (f) Subcellular localization of RHC1 inArabidopsismesophyll protoplasts.35S::RHC1–GFP,35S::SLAC1–GFPand35S::GFPwere transiently expressed inArabidopsismesophyll protoplasts, respectively. SLAC1–GFP fusion was used as a control for plasma membrane localization and GFP alone was used as a control for cytosol and nuclear localization. Scale bars, 5 μm. (g) Time courses of stomatal conductance in response to changes in CO2concentration in wild-type (WT),rhc1mutants and a complementation line (comp). Stomatal conductance was measured using a gas-exchange system. The leaves were stabilized in 400 p.p.m. CO2before changing to 800 p.p.m. CO2. Values of stomatal conductance at 400 p.p.m. CO2were normalized to 1. (n=5 leaves forrhc1,n=4 for WT andn=3 for the complemented line.) Data are presented as means±s.e.m. (h) High [CO2]-induced stomatal closing is impaired inrhc1mutant leaf epidermis. Leaf epidermis were treated with 800 p.p.m. CO2for 30 min (n=3 experiments, 60 stomata per condition, genotype blind analyses; *P<0.001, pairwise Student’st-test). (i) Stomata inrhc1leaves close in response to abscisic acid (ABA). Leaf epidermis were treated with 0, 1, 10 and 50 μM ABA for 30 min (n=3 experiments, 60 stomata per condition). (j) Stomata inrhc1leaves close in response to CaCl2. Leaf epidermis were treated with 0, 2 and 10 mM CaCl2for 120 min (n=3 experiments, 60 stomata per condition). Data inh–jare presented as means±s.e.m. Figure 1: The rhc1 mutant plants are defective in stomatal responses to CO 2 . ( a – e ) Expression of RHC1::GUS in leaves ( a ), flowers ( b ), vascular systems ( c ), stem ( d ) and guard cells ( e ). Scale bars, 500 μm ( a , b ), 100 μm ( c , d ), 5 μm ( e ). ( f ) Subcellular localization of RHC1 in Arabidopsis mesophyll protoplasts. 35S::RHC1–GFP , 35S::SLAC1–GFP and 35S::GFP were transiently expressed in Arabidopsis mesophyll protoplasts, respectively. SLAC1–GFP fusion was used as a control for plasma membrane localization and GFP alone was used as a control for cytosol and nuclear localization. Scale bars, 5 μm. ( g ) Time courses of stomatal conductance in response to changes in CO 2 concentration in wild-type (WT), rhc1 mutants and a complementation line (comp). Stomatal conductance was measured using a gas-exchange system. The leaves were stabilized in 400 p.p.m. CO 2 before changing to 800 p.p.m. CO 2 . Values of stomatal conductance at 400 p.p.m. CO 2 were normalized to 1. ( n =5 leaves for rhc1 , n =4 for WT and n =3 for the complemented line.) Data are presented as means±s.e.m. ( h ) High [CO 2 ]-induced stomatal closing is impaired in rhc1 mutant leaf epidermis. Leaf epidermis were treated with 800 p.p.m. CO 2 for 30 min ( n =3 experiments, 60 stomata per condition, genotype blind analyses; * P <0.001, pairwise Student’s t -test). ( i ) Stomata in rhc1 leaves close in response to abscisic acid (ABA). Leaf epidermis were treated with 0, 1, 10 and 50 μM ABA for 30 min ( n =3 experiments, 60 stomata per condition). ( j ) Stomata in rhc1 leaves close in response to CaCl 2 . Leaf epidermis were treated with 0, 2 and 10 mM CaCl 2 for 120 min ( n =3 experiments, 60 stomata per condition). Data in h – j are presented as means±s.e.m. Full size image Stomatal pores allow influx of atmospheric CO 2 in exchange for transpirational water loss. Stomatal aperture is highly regulated by light, CO 2 concentration and the phytohormone ABA [5] , [13] , [43] , [44] . The CO 2 -resistant growth of rhc1 mutant plants together with guard cell expression of RHC1 gene suggests that RHC1 may function in stomatal response to CO 2 . We thus compared the WT and the rhc1 mutant plants in their stomatal responses using the transpiration assay [45] . Increasing CO 2 concentration from 400 to 800 p.p.m. reduced stomatal conductance effectively in the WT, whereas rhc1 plants showed a greatly reduced response ( Fig. 1g ). These differences in stomatal conductance were not a result of variation in stomatal number, because rhc1 and WT leaves have similar stomatal density ( Supplementary Fig. 4 ). We also examined the stomatal aperture of detached leaves exposed to high CO 2 . After exposure to elevated CO 2 levels, stomatal aperture was reduced in the WT plants, but not in the rhc1 mutant ( Fig. 1h ), consistent with the stomatal conductance results in Fig. 1g . To determine whether RHC1 is involved in other guard-cell signal transduction pathways, we assayed stomatal apertures in response to ABA and Ca 2+ and found no difference between rhc1 mutant and WT plants ( Fig. 1i,j ). RHC1 functions upstream of HT1 Several components have been identified as specific regulators in CO 2 response in guard cells, which include CAs and HT1 that function as a positive and negative regulator, respectively. The ca1ca4 and ht1 mutants showed impaired CO 2 regulation of stomatal movements, but retained normal ABA response. As RHC1 also functions specifically in the CO 2 response pathway, we examined a possible relationship among RHC1, CAs and HT1. We first performed a bimolecular fluorescence complementation (BiFC) assay in Arabidopsis protoplasts [46] , [47] . The combination of RHC1-nVenus and CA4-cCFP or RHC1-nVenus and HT1-cCFP produced a green fluorescent signal in the plasma membrane ( Fig. 2a ), indicating that RHC1 can interact with CA4 and HT1 in the plasma membrane in plant cells. The OST1 protein kinase, a positive regulator of ABA and CO 2 signalling pathways, showed no interaction with RHC1 ( Fig. 2a ), suggesting that interaction of RHC1 with CAs and HT1 was specific. To test the interaction between CA1/4 and RHC1 by an alternative approach, and further identify the regions responsible for interaction, we expressed recombinant proteins in Escherichia coli and performed pull-down assays. The glutatione S -transferase (GST)-fusion proteins containing the N- or C-terminal cytosolic domain of the RHC1 were incubated with His-tagged CA4, and the co-purified proteins were analysed by SDS–polyacrylamide gel electrophoresis (PAGE). Both the N terminus and C terminus of the RHC1 protein were co-purified with CA4 ( Fig. 2b ). In contrast, no CA4-His enrichment was observed when GST was incubated with CA4-His. These data provide further support for the physical interaction between RHC1 and CA enzymes. Then the interaction of RHC1 and HT1 was alternatively confirmed by split-ubiquitin yeast two-hybrid (Y2H) analysis [48] ( Fig. 2c ). We next examined the genetic interaction of RHC1 and HT1 using double-mutant analysis. Our results showed that rhc1 ht1-2 double-mutant plants exhibited a constitutive high CO 2 response similar to ht1-2 plants, indicating that HT1 is epistatic to RHC1 ( Fig. 2d,e ). In other words, RHC1 functions upstream of HT1 in the CO 2 response pathway. 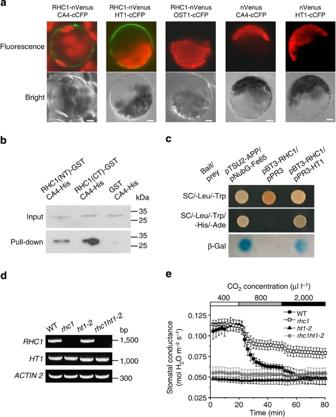Figure 2: RHC1 physically interacts with CAs and HT1 and functions upstream of HT1. (a) RHC1 interaction with CA4 and HT1 as assayed in BiFC usingArabidopsismesophyll protoplasts. Protoplasts were transfected with different combinations of expression vectors encoding RHC1-nVenus, CA4-cCFP, HT1-cCFP, OST1-cCFP, nVenus or cCFP. Scale bars, 5 μm. (b) GST pull-down assay. Immobilized GST, or RHC1 N- or C-terminal region fused to GST (RHC1(NT)–GST or RHC1(CT)–GST, respectively) was incubated with his-tagged CA4 (CA4-His). After washing, CA4 bound to fusion proteins was eluted and resolved by SDS–PAGE and visualized by western blot analysis with anti-His antibody. (c) Interaction of RHC1 and HT1 in a yeast-based split-ubiquitin system. pTSU2-APP/pNubG-Fe65 and pBT3-RHC1/pPR3 were used as positive and negative controls, respectively. (d) Selection ofrhc1ht1-2double-mutant. Gel image shows genotyping by PCR of WT,rhc1,ht1-2andrhc1ht1-2plants. (e) Time-resolved stomatal conductance analyses in WT,rhc1,ht1-2andrhc1 ht1-2double-mutant leaves in response to changes of CO2concentrations (n=3). The data represent means±s.e.m. Figure 2: RHC1 physically interacts with CAs and HT1 and functions upstream of HT1. ( a ) RHC1 interaction with CA4 and HT1 as assayed in BiFC using Arabidopsis mesophyll protoplasts. Protoplasts were transfected with different combinations of expression vectors encoding RHC1-nVenus, CA4-cCFP, HT1-cCFP, OST1-cCFP, nVenus or cCFP. Scale bars, 5 μm. ( b ) GST pull-down assay. Immobilized GST, or RHC1 N- or C-terminal region fused to GST (RHC1(NT)–GST or RHC1(CT)–GST, respectively) was incubated with his-tagged CA4 (CA4-His). After washing, CA4 bound to fusion proteins was eluted and resolved by SDS–PAGE and visualized by western blot analysis with anti-His antibody. ( c ) Interaction of RHC1 and HT1 in a yeast-based split-ubiquitin system. pTSU2-APP/pNubG-Fe65 and pBT3-RHC1/pPR3 were used as positive and negative controls, respectively. ( d ) Selection of rhc1 ht1-2 double-mutant. Gel image shows genotyping by PCR of WT, rhc1 , ht1-2 and rhc1 ht1-2 plants. ( e ) Time-resolved stomatal conductance analyses in WT, rhc1 , ht1-2 and rhc1 ht1-2 double-mutant leaves in response to changes of CO 2 concentrations ( n =3). The data represent means±s.e.m. Full size image RHC1 is required for activation of the S-type channels Previous studies have shown that during CO 2 -induced stomatal closure, CO 2 is first catalysed by CAs into bicarbonate, and elevated bicarbonate in turn activates the S-type anion channels through unknown signalling events, among which HT1 kinase acts as a negative regulator downstream of HCO 3 − production and upstream of the S-type anion channel activation [18] . Our earlier results showed that RHC1 interacts with and functions upstream of HT1. If RHC1–HT1 interaction indeed serves as a missing link upstream of anion channel activation, RHC1 should be required for high-HCO 3 − -induced activation of the S-type anion channels in guard cells. Hence, we investigated the effect of RHC1 disruption on bicarbonate activation of the S-type anion channels in guard cells by whole-cell patch-clamp recording. The results showed that bicarbonate activation of the S-type anion channels was strongly impaired in guard cells from rhc1 mutant plants, as compared with the WT. At −145 mV in the presence of 13.5 mM HCO 3 − , the current amplitude in rhc1 guard cells was −31.9±3.4 pA (mean±s.e.m. ; n =8), compared with −54.4±9.5 pA (mean±s.e.m. ; n =5) in the WT ( Fig. 3a,b ). However, in the rhc1ht1-2 double-mutant, bicarbonate activation of the S-type anion channels was restored to the WT level ( Fig. 3a,b ), indicating that RHC1 acts as an upstream repressor of the negative regulator HT1. 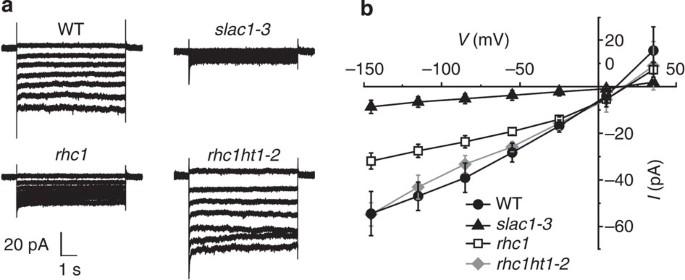Figure 3: RHC1 is required for bicarbonate activation of S-type anion channels inArabidopsisguard cells. (a) Patch-clamp whole-cell recordings with 13.5 mM total bicarbonate added to the pipette solution in wild-type,slac1-3,rhc1andrhc1ht1-2guard cell protoplasts. (b) Steady-state current–voltage relationships of recordings as ina. The data are presented as means±s.e.m. (wild type,n=5;slac1-3,n=4;rhc1,n=8;rhc1 ht1-2,n=5). Figure 3: RHC1 is required for bicarbonate activation of S-type anion channels in Arabidopsis guard cells. ( a ) Patch-clamp whole-cell recordings with 13.5 mM total bicarbonate added to the pipette solution in wild-type, slac1-3 , rhc1 and rhc1 ht1-2 guard cell protoplasts. ( b ) Steady-state current–voltage relationships of recordings as in a . The data are presented as means±s.e.m. (wild type, n =5; slac1-3 , n =4; rhc1 , n =8; rhc1 ht1-2 , n =5). Full size image HT1 prevents OST1-induced activation of SLAC1 If RHC1 is an upstream component of HT1, how does HT1 exert its negative effect on SLAC1? A recent study showed that OST1 loss-of-function mutants are strongly impaired in CO 2 -induced stomatal closing and in HCO 3 − activation of the S-type anion channels [16] . This finding indicates that OST1, a protein kinase that regulates SLAC1 activity in the ABA pathway, may be a central integrator of CO 2 and ABA signal transduction in the regulation of SLAC1 in guard cells. While the ABA signal connects to OST1 through ABA receptors and 2C-type protein phosphatases [5] , [49] , it is not known how the CO 2 signal is linked to OST1. We thus tested the possibility that OST1 may serve as a downstream target of HT1. First, we conducted a BiFC assay and found that HT1 and OST1 interacted with each other in Arabidopsis protoplasts ( Fig. 4a ). Then, we performed in vitro kinase assays and found that HT1 phosphorylated OST1, but OST1 did not phosphorylate HT1 ( Fig. 4b ). Using the N terminus of SLAC1 (SLAC1-NT; amino acids 1–186) as the substrate of OST1 kinase [23] , [24] , we found that the kinase activity of OST1 was inhibited when HT1 was present, whereas HT1 kinase did not phosphorylate SLAC1-NT in the same assay, and the kinase-inactive variant of HT1 (K113W) [13] did not affect the OST1 activity against SLAC1-NT ( Fig. 4b ). Taken together, the results indicate that HT1 interacts with and phosphorylates OST1 thereby inhibiting the kinase activity of OST1 against SLAC1. We further performed two-electrode voltage-clamp experiments to examine how the SLAC1 channel may be regulated by the upstream kinases OST1 and HT1. Co-expression of SLAC1 and OST1 kinase significantly activated the SLAC1 channel ( Fig. 4c,d ), consistent with previous results [23] , [24] . Co-expressing HT1 with SLAC1 did not alter SLAC1 activity ( Fig. 4c,d ). When we co-expressed SLAC1, OST1 and HT1 in oocytes, however, we found that anion currents activated by OST1 were abolished ( Fig. 4c,d ). The kinase-inactive variant of HT1 (K113W) did not affect OST1-activated SLAC1 anion currents ( Fig. 4c,d ), indicating that phosphorylation of OST1 by HT1 is essential in this regulation. As a control, we included another protein kinase, CPK3, which has no significant effect on SLAC1 refs 30 , 31 , 32 , that did not inhibit OST1-activated SLAC1 anion currents ( Fig. 4c,d ), demonstrating that the inhibition of HT1 on OST1 was specific. Further, we produced the ht1-2ost1 double-mutant by crossing the single mutants and compared their behaviour in CO 2 response. We found that the double-mutant is impaired in high-CO 2 -induced stomatal closing, similar to ost1 single mutant [18] , indicating that OST1 is downstream of HT1 kinase in the pathway ( Fig. 4e ), consistent with the conclusion deduced from the biochemical and electrophysiological assays presented earlier ( Fig. 4a–d ). 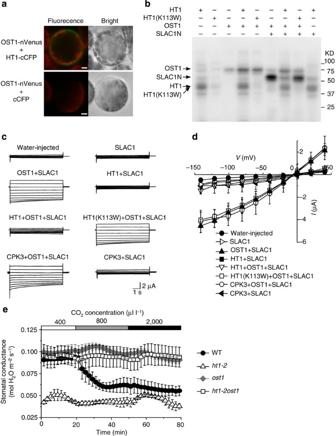Figure 4: HT1 phosphorylates OST1 and prevents the activation of SLAC1 by OST1. (a) HT1 interaction with OST1 in the BiFC assay. Co-expression of OST1-nVenus and cCFP was used as control. Scale bars, 5 μm. (b) HT1 phosphorylates OST1 and inhibits the phosphorylation of SLAC1 by OST1. HT1(K113W) is a kinase-dead mutant. SLAC1N: the cytosolic N terminus of SLAC1. (c) Whole-cell recordings from oocytes co-expressing SLAC1, OST1, HT1 (or HT1 mutant K113W) or CPK3. (d) Steady-stateI–Vrelationships of recordings as inc. The data are presented as means±s.d. (water-injected,n=12; SLAC1,n=12; OST1+SLAC1,n=12; HT1+SLAC1,n=13; HT1+OST1+SLAC1,n=13; HT1(K113W)+OST1+SLAC1,n=13, CPK3+OST1+SLAC1,n=12; CPK3+SLAC1,n=12). (e) Time-resolved stomatal conductance analyses in WT,ht1-2,ost1andht1-2 ost1double-mutant leaves in response to changes of CO2concentrations (WT,n=3;ht1-2,n=3;ost1,n=5;ht1-2 ost1,n=5). The data represent means±s.e.m. Figure 4: HT1 phosphorylates OST1 and prevents the activation of SLAC1 by OST1. ( a ) HT1 interaction with OST1 in the BiFC assay. Co-expression of OST1-nVenus and cCFP was used as control. Scale bars, 5 μm. ( b ) HT1 phosphorylates OST1 and inhibits the phosphorylation of SLAC1 by OST1. HT1(K113W) is a kinase-dead mutant. SLAC1N: the cytosolic N terminus of SLAC1. ( c ) Whole-cell recordings from oocytes co-expressing SLAC1, OST1, HT1 (or HT1 mutant K113W) or CPK3. ( d ) Steady-state I – V relationships of recordings as in c . The data are presented as means±s.d. (water-injected, n =12; SLAC1, n =12; OST1+SLAC1, n =12; HT1+SLAC1, n =13; HT1+OST1+SLAC1, n =13; HT1(K113W)+OST1+SLAC1, n =13, CPK3+OST1+SLAC1, n =12; CPK3+SLAC1, n =12). ( e ) Time-resolved stomatal conductance analyses in WT, ht1-2 , ost1 and ht1-2 ost1 double-mutant leaves in response to changes of CO 2 concentrations (WT, n =3; ht1-2 , n =3; ost1 , n =5; ht1-2 ost1 , n =5). The data represent means±s.e.m. Full size image Reconstitution of SLAC1 activation by HCO 3 − in oocytes Thus far, we have shown that RHC1 interacts with HT1 and functions upstream of HT1 ( Fig. 2a,c–e ). HT1 phosphorylates OST1 and inhibits OST1-mediated activation of SLAC1 ( Fig. 4 ). Furthermore, RHC1 also physically interacts with CAs ( Fig. 2a,b ). On the basis of these results, we hypothesized that the high concentration of HCO 3 − generated by CAs may be perceived by RHC1 that in turn interacts with HT1 to remove its negative effect on SLAC1 activation. To test this possibility, we attempted to reconstitute the molecular relay in oocytes using SLAC1 activity as an assay. When RHC1, HT1, OST1 and SLAC1 were co-expressed in the oocytes, SLAC1 was inactive without HCO 3 − (or with low levels of HCO 3 − ), mimicking the low-CO 2 condition in the guard cells ( Fig. 5a,b ). However, when high levels of HCO 3 − (6.75 or 13.5 mM HCO 3 − ) was injected into the oocytes expressing the RHC1–HT1–OST1–SLAC1 module, SLAC1 was activated ( Fig. 5a,b ). When 13.5 mM HCO 3 − was injected into oocytes expressing HT1, OST1 and SLAC1 (without RHC1), SLAC1 remained inactive ( Fig. 5a,b ). In the oocyte expressing RHC1, OST1 and SLAC1 (without HT1), SLAC1 was activated independent of HCO 3 − ( Fig. 5a,b ). These results show that RHC1 perceives HCO 3 − and removes the inhibitory effect of HT1 on SLAC1 activation by OST1. 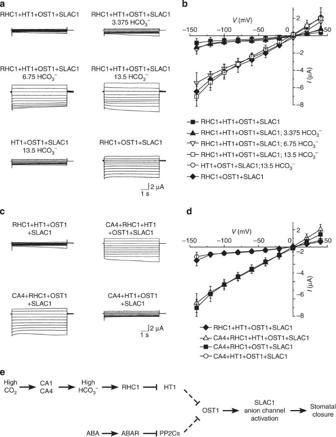Figure 5: Reconstitution of the CO2-sensing pathway for SLAC1 activation in oocytes. (a) Bicarbonate-dependent activation of SLAC1 requires RHC1. Whole-cell recording of SLAC1 activity in oocytes co-expressing SLAC1 with different combinations of signalling components RHC1, HT1 and OST1. Anion currents were recorded from the oocytes injected with different concentrations of HCO3−. (b) Steady-stateI–Vrelationships of recordings as ina. The data are presented as means±s.d. (RHC1+HT1+OST1+SLAC1,n=12; RHC1+HT1+OST1+SLAC1; 3.375 HCO3−,n=15; RHC1+HT1+OST1+SLAC1; 6.75 HCO3−,n=11; RHC1+HT1+OST1+SLAC1; 13.5 HCO3−,n=10; HT1+OST1+SLAC1; 13.5 HCO3−,n=14; RHC1+OST1+SLAC1,n=12). (c) Bicarbonate activation of SLAC1 in oocytes co-expressing combinations of not only those signalling components inabut including CA as well. (d) Steady-stateI–Vrelationships of recordings as inc. The data are presented as means±s.d. (RHC1+HT1+OST1+SLAC1,n=10; CA4+RHC1+HT1+OST1+SLAC1,n=11; CA4+RHC1+OST1+SLAC1,n=10; CA4+HT1+OST1+SLAC1,n=10). (e) A working model for a rapid calcium-independent CO2signal pathway inArabidopsisguard cells. The details of this working model are described in the text. Figure 5: Reconstitution of the CO 2 -sensing pathway for SLAC1 activation in oocytes. ( a ) Bicarbonate-dependent activation of SLAC1 requires RHC1. Whole-cell recording of SLAC1 activity in oocytes co-expressing SLAC1 with different combinations of signalling components RHC1, HT1 and OST1. Anion currents were recorded from the oocytes injected with different concentrations of HCO 3 − . ( b ) Steady-state I – V relationships of recordings as in a . The data are presented as means±s.d. (RHC1+HT1+OST1+SLAC1, n =12; RHC1+HT1+OST1+SLAC1; 3.375 HCO 3 − , n =15; RHC1+HT1+OST1+SLAC1; 6.75 HCO 3 − , n =11; RHC1+HT1+OST1+SLAC1; 13.5 HCO 3 − , n =10; HT1+OST1+SLAC1; 13.5 HCO 3 − , n =14; RHC1+OST1+SLAC1, n =12). ( c ) Bicarbonate activation of SLAC1 in oocytes co-expressing combinations of not only those signalling components in a but including CA as well. ( d ) Steady-state I – V relationships of recordings as in c . The data are presented as means±s.d. (RHC1+HT1+OST1+SLAC1, n =10; CA4+RHC1+HT1+OST1+SLAC1, n =11; CA4+RHC1+OST1+SLAC1, n =10; CA4+HT1+OST1+SLAC1, n =10). ( e ) A working model for a rapid calcium-independent CO 2 signal pathway in Arabidopsis guard cells. The details of this working model are described in the text. Full size image CAs facilitate the conversion of CO 2 into bicarbonate and physically interact with RHC1 at plasma membrane, which may cause a local increase in bicarbonate in the vicinity of the CA–RHC1 interaction ( Fig. 2a,b ). We co-expressed CA4, RHC1, HT1, OST1 and SLAC1 in oocytes and found that SLAC1 was activated ( Fig. 5c,d ). When CA4, HT1, OST1 and SLAC1 (without RHC1) were co-expressed, SLAC1 was inactive ( Fig. 5c,d ), indicating that RHC1 serves as a bridging component between CAs and HT1, providing a functional relevance of CA–RHC1 interaction. In the oocyte expressing CA4, RHC1, OST1 and SLAC1 (without HT1), SLAC1 was constitutively active ( Fig. 5c,d ). These findings support the model that CAs function as a first step in producing elevated HCO 3 − under high CO 2 , and RHC1 acts as a HCO 3 − -sensing component to overcome HT1 inhibition of the downstream signalling events leading to SLAC1 anion channel activation. Previous studies have shown that CA-mediated elevation in HCO 3 − is required for activation of SLAC1 anion channels in Arabidopsis guard cells, leading to stomatal closure [5] , [20] . However, HCO 3 − does not activate SLAC1 directly [18] , [23] , leaving a gap in the signalling pathway. Our study here identified RHC1, a MATE-type protein, as the bridging regulator downstream of HCO 3 − in the CO 2 signalling pathway based on the following results: (1) RHC1 interacts with and functions downstream of CAs that converts CO 2 into HCO 3 − ( Fig. 2a,b ), supporting its position as an immediate component following CAs; (2) RHC1 acts upstream of HT1, a negative regulator of CO 2 response, and overcomes its negative effect on SLAC1 activation ( Figs 2a,c–e and 3 ); (3) RHC1 is essential for SLAC1 activation by elevated HCO 3 − in planta ( Fig. 3 ); (4) using CA, RHC1, HT1, OST1 and SLAC1, we successfully reconstituted the molecular pathway for CO 2 -sensing in oocytes, and RHC1 bridges the gap between CA and HT1 as a required element for HCO 3 − -dependent activation of SLAC1 ( Fig. 5 ). Taken together, we propose that RHC1 functions as a HCO 3 − -sensing component in the CO 2 signalling pathway in Arabidopsis guard cells. Because RHC1 is a member of the MATE-type transporter family [41] , [42] , it will be important to determine whether RHC1 has transporter activity and whether this activity is related to CO 2 sensing. We noted that stomatal movements in rhc1 mutant plants are not completely insensitive to changes in CO 2 concentration ( Fig. 1g,h ), suggesting presence of other RHC1-like HCO 3 − -sensing components either in the MATE family or in other protein families in Arabidopsis . Further studies should be directed to dissect the detailed molecular mechanism of how RHC1 works and to identify other HCO 3 − -sensing components. Discovery of RHC1 not only placed a new component into the CO 2 signalling pathway, it also prompted us to explore the relationship of ABA and CO 2 signal transduction in Arabidopsis . Specifically, we identified a mechanism for the regulation of OST1 by CO 2 . As a key positive regulator of ABA response, OST1 is subject to negative regulation by group-A protein phosphatase type 2Cs (PP2C) [50] , [51] . Group-A PP2Cs interact physically with OST1, and efficiently inactivate OST1 via dephosphorylation of multiple Ser/Thr residues in the activation loop [50] , [51] . Here, we identified a different mechanism for the inactivation of OST1 in CO 2 response, namely, inhibition through phosphorylation by HT1 kinase ( Fig. 4 ). This finding clearly positions OST1 at the convergence point of ABA and CO 2 signalling pathways. Further research on the structural basis for the HT1–OST1 interaction and phosphorylation sites on OST1 will provide a more detailed molecular mechanism underlying OST1 inhibition by HT1 kinase. Given SLAC1 is also regulated by other protein kinases including CPKs [30] , [31] , [32] and calcium sensor kinases CBL-CIPKs [52] , further work should also be conducted to find out whether HT1, similar to the PP2C A-type phosphatases in ABA signalling, can also interact with and inhibit calcium-dependent kinases. We propose a working model for a rapid calcium-independent CO 2 signalling pathway leading to stomatal closure ( Fig. 5e ). When the atmospheric CO 2 concentration is low, the intracellular HCO 3 − concentration is also low. In this case, HT1 interacts with and phosphorylates OST1, inhibiting OST1 activity. SLAC1 is inactive and stomata remain open. Under high CO 2 concentrations, CAs produce elevated intracellular HCO 3 − that in turn causes conformational change of RHC1 enhancing its interaction with HT1. Physical interaction of RHC1 and HT1 recruits HT1 to the plasma membrane. This switch breaks down the HT1–OST1 interaction and relieves inhibition of OST1 kinase by HT1. The active OST1 subsequently phosphorylates and activates SLAC1 to initiate anion efflux, triggering the closure of stomatal pores. Plant materials and growth conditions All Arabidopsis lines used in this study were derived from the Columbia (Col-0) ecotype. Under normal growth conditions, plants were grown in a growth chamber at 22 °C, 65–80% humidity and a 16-h-light/8-h-dark regime at ~75 μmol m −2 s −1 . For high [CO 2 ] treatment, a similar growth chamber was equipped with an automatic CO 2 control unit that maintained the CO 2 concentration at 700 or 800 p.p.m., other conditions remained the same. T-DNA mutants (SALK_123674) were obtained from the Arabidopsis Biological Resource Centre ( www.arabidopsis.org ). Cloning procedures For the GUS-staining assay, Col-0 genomic DNA was used as a template for the amplification of the promoter of the RHC1 gene. A 1.7 kb fragment upstream of the gene was cloned into pBI101.1 vector using RHC1 promoter primers. To complement rhc1 mutant, the ProRHC1::RHC1 was cloned into pCAMBIA 1300 vector. For the subcellular localization assay, complementary DNAs (cDNAs) of Arabidopsis RHC1 and SLAC1 encoding full-length proteins were PCR-amplified with gene-specific primers. The resulting cDNAs were inserted into pCAMBIA 1302 to produce the 35S::RHC1 (or SLAC1 )– GFP constructs. For BiFC in Arabidopsis mesophyll protoplasts, the full-length RHC1 , OST1 , HT1 and CA4 were subcloned into pSAT1-nVenus-N (or pSAT1-cCFP-N) [46] to produce 35S::RHC1-nVenus , 35S::OST1-cCFP , 35S::HT1-cCFP , 35S:: CA4-cCFP and 35S::OST1-nVenus with gene-specific primers. For two-electrode voltage-clamp analysis in Xenopus oocytes, RHC1 , HT1 , HT1(K133W) , SLAC1 , CA4 , OST1 and CPK3 cDNAs encoding full-length proteins were inserted into pGEMHE with gene-specific primers. For in vitro pull-down and kinase assays, cDNAs of RHC1 (NT 1–36AA), RHC1 (CT 458–491AA), SLAC1 (NT 1–186AA) and CA4 were inserted into pGEX4T-1 vector to produce GST–RHC1(NT) , GST–RHC1(CT) and GST–CA4 constructs. HT1 cDNAs encoding full-length WT or mutant proteins were inserted into pET28a to produce the His-HT1 and His-HT1(K133W) with gene-specific primers. For yeast split-ubiquitin analysis, the coding sequence of RHC1 or HT1 was cloned into the pBT3-N/pPR3-N vector (Dualsystems Biotech), to yield plasmids pBT3-N-RHC1 and pPR3-N-HT1. The primers used are summarized in Supplementary Table 1 . RNA extraction and reverse transcription–PCR Total RNA was isolated from leaves of WT or mutant plants using Trizol reagent (Invitrogen). One μg of RNA was reverse-transcribed with Superscript Ш (Invitrogen) following the manufacturer’s instructions. The cDNA was used as a template for amplification. The primers used are listed in Supplementary Table 1 . Arabidopsis ACTIN 2 was amplified as an endogenous reference for normalization. GUS staining The construct of ProRHC1::GUS was transformed into agrobacterium GV3101 and further transformed into WT Arabidopsis plants [53] . Histochemical staining for GUS activity was performed as described previously [14] . In detail, tissues from the T2 transgenic plants were collected in Eppendorf tubes and placed in cold 90% acetone on ice and then fixed at room temperature for 30 min. The samples were rinsed with cold staining buffer without X-Gluc. Then, the staining buffer was removed from samples and staining buffer was added with 2 mM X-Gluc on ice and incubated for 12 h at 37 °C. After staining, staining buffer was removed and the samples were destained with 70% ethanol until tissues were clear. The observed staining patterns were recorded with a microscope (Nikon SMZ1500). Protoplast isolation and transformation Arabidopsis plants grow under 13 h light/11 h dark for 3–4 weeks; well expanded leaves are used to isolated protoplasts. Isolation and transient protoplast transformation was performed as described previously [54] . Briefly, leaves were sliced on a paper and immediately transferred into enzyme solution, the digestion was continued for about 3 h with gentle shaking in the dark. After incubation, the enzyme solution containing protoplasts was filtered, then washing solution was added and protoplasts were collected by centrifugation and resuspended in MMG solution. After polyethylene glycol (PEG)-mediated transfection, protoplasts were incubated at 25 °C in the dark for 24 h. Subcellular localization The expression constructs 35S::RHC1 , 35S::SLAC1 – GFP or 35S::GFP were transformed into Arabidopsis protoplasts by PEG-mediated transfection [54] . Protoplasts were stained with 2 μM FM4-64 dye for 5 min to stain the plasma membrane. Protoplast images were taken by confocal microscopy (Zeiss 5-LIVE) operated with LSM Image Browser software. Gas exchange and stomatal aperture measurements Stomatal conductance recordings from intact, mature non-senescent leaves of 5–7-week-old plants were conducted using a Li-6400 infrared (IRGA)-based gas-exchange analyser with a fluorometer chamber (Li-Cor Inc.) [17] . Temperature and relative humidity were held at 20 °C and ~60–70%, respectively. For analysing stomatal responses to different CO 2 concentrations, photon flux density was 75 μmol m −2 s −1 . The leaves were stabilized in 400 p.p.m. CO 2 before changing to 800 p.p.m. CO 2 . Leaves were exposed to 800 p.p.m. CO 2 , 2,000 p.p.m. CO 2 and 400 p.p.m. CO 2 for 30 min in each condition. Values of stomatal conductance at 400 p.p.m. CO 2 were normalized to 1. For responses to light/dark transitions, leaves were kept at a constant CO 2 concentration of 400 p.p.m. The leaves were stabilized in 130 μmol m −2 s −1 before changing to 0 μmol m −2 s −1 . Light and dark periods were switched every 30 min. Values of stomatal conductance at 130 μmol m −2 s −1 were normalized to 1. For stomatal aperture measurements in response to CO 2 , leaf epidermal layers were pre-incubated for 2.5 h in pre-incubation buffer (10 mM MES, 10 mM KCl, 50 μM CaCl 2 at pH 6.15) (initial apertures) and then treated with 800 p.p.m. CO 2 for 30 min under white light (200 μmol m −2 s −1 ). Stomatal apertures were analysed only in stomatal complexes with no mesophyll cells in their vicinity. For responses to ABA and CaCl 2 , intact leaf epidermis were incubated for 3 h in stomatal opening buffer (5 mM MES, 10 mM KCl, 50 μM CaCl 2 , pH 5.6), and exposed to ABA (0, 1, 10 and 50 μM) and CaCl 2 (0, 2 and 10 mM). Thereafter stomatal apertures were measured [16] . BiFC experiments The indicated pairs of expression constructs [46] were co-transformed into Arabidopsis mesophyll protoplasts by PEG-mediated transfection [54] . Protoplast images were taken by confocal microscopy (Zeiss 5-LIVE) operated with LSM Image Browser software. Purification of fusion proteins in E. coli GST -tagged RHC1 (NT) , RHC1 (CT) , OST1 and SLAC1 (NT) in the pGEX-KG vector and His -tagged CA4 , HT1 and HT1(K133W) in the pET28a vector were induced by 1 mM isopropyl-β- D -thiogalactoside in E. coli strain BL21 (DE3) and purified by a standard procedure. Briefly, for GST-tag fusion proteins purification, bacteria were lysed in PBS containing 1% Triton X-100, 1 mM phenylmethylsulphonyl fluoride and a proteinase inhibitor cocktail by sonification, and GST-fusion proteins were purified using glutathione agarose beads (GE Healthcare). For His-tag fusion proteins, bacteria were lysed in lysis buffer containing 50 mM NaH 2 PO 4 , 300 mM NaCl, 10 mM imidazole, 0.05% Tween 20, 1 mM phenylmethylsulphonyl fluoride and a proteinase inhibitor cocktail, and His-fusion proteins were purified using Ni-NTA Magnetic Agarose Beads (QIAGEN). GST pull-down assay Purified GST-tagged RHC1(NT), RHC1(CT) and GST (2 μg each) were incubated with 20 μl glutathione agarose beads in PBS buffer at 4 °C for 2 h with constant rotation. Then each sample was centrifuged and the supernatants were removed, 1 ml cell lysates containing equal amount of His-tagged CA4 protein was added and rotated for another 4 h at 4 °C. After co-incubation, washed the agarose 6 times with PBS buffer and then subjected to SDS–PAGE and western blot analysis, the His-tagged CA4 was detected with an anti-His antibody (abcam, ab18184, 1:1,000 dilution). Uncropped blots are shown in Supplementary Fig. 5 . Yeast two-hybrid assays Plasmids for Y2H assays were introduced into yeast strain NMY51 by the lithium acetate method [55] . β-galactosidase activity was determined using filter assays [56] . Cells were streaked on filter paper, then frozen briefly in liquid nitrogen, defrosted and placed in Petri dishes filled with 0.5% agarose containing 35 mM β-mercaptoethanol (v/v) and 1.5 mg ml −1 of 5-bromo-4-chloro-3-indolyl-β- D -galactoside (Sigma). Patch-clamp whole-cell recording from guard cell protoplasts Arabidopsis guard cell protoplasts were isolated enzymatically from leaf epidermal strips of 4–6-week-old plants. Arabidopsis rosette leaves were blended in a commercial blender in deionized water three times for 5 s each and collected using a nylon mesh (pore size, 62 μm). The collected epidermal tissue was incubated in 10 ml of medium containing 1% Cellulase R-10, 0.5% Macerozyme R-10 (Yakult), 0.5% bovine serum albumin, 0.5 M mannitol, 0.1 mM KCl, 0.1 mM CaCl 2 , 10 mM ascorbic acid and 0.1% kanamycin sulfate, pH 5.5 (with KOH), for 15–17 h at 24 °C on a shaker. Then isolated guard cell protoplasts were collected. Whole-cell patch-clamp recordings were made using a MultiClamp 700B amplifier (Axon Instruments). Patch pipettes were pulled from borosilicate glass on a P-97 horizontal puller (Sutter Instruments). Giga ohm seals between electrode and plasma membrane (>10 GΩ) were obtained by suction. Cells were pulled up to the bath solution surface to reduce stray capacitance. Whole-cell configurations were established by applying increased suction to the interior of the pipette. For analyses of intracellular bicarbonate/CO 2 activation of S-type anion currents [17] , [18] , the pipette solution contained 150 mM CsCl, 2 mM MgCl 2 , 6.7 mM ethylene glycol tetraacetic acid (EGTA), 5 mM Mg-adenosine triphosphate, 5 mM Tris-guanosine triphosphate, 6.03 mM CaCl 2 (2 μM free Ca 2+ ), 13.5 mM CsHCO 3 (11.5 mM HCO 3 − and 2 mM free CO 2 ) and 1 mM HEPES/Tris (pH 7.1). CsHCO 3 was dissolved in the pipette solution right before patch-clamp experiments and pH was adjusted to the indicated values. The pipette solution was stored using air-tight precision glass syringes during patch-clamp experiments to prevent CO 2 equilibration with the surrounding air. The concentrations of bicarbonate and free CO 2 in solutions were calculated using the Henderson–Hasselbalch equation (pH=pK1+log[HCO 3 − ]/[CO 2 ]) [18] , [57] . [HCO 3 − ] represents the free bicarbonate concentration; [CO 2 ] represents the free CO 2 concentration. A value pK 1 =6.352 was used for calculations. The bath solution contained 30 mM CsCl, 2 mM MgCl 2 , 5 mM CaCl 2 and 10 mM Mes/Tris at pH 5.6. During recordings of S-type anion currents, the membrane voltage was stepped to potentials starting at +35 to −145 mV for 7 s with −30 mV decrements and the holding potential was +30 mV. The inter-pulse period was 5 s. Liquid junction potentials were determined using Clampex 10.2. No leak subtraction was applied for all current–voltage curves. Steady-state currents were the average currents during the last 500 ms of pulses. In vitro kinase assay The in vitro kinase assays were performed as previously described [13] , [23] , [24] . The in vitro kinase buffer consisted of 25 mM Tris, pH 7.5, 10 mM MgCl 2 and 1 mM CaCl 2 , a cocktail of protease inhibitors and 5 μCi [γ- 32 P] adenosine tri-phosphate. Reactions were carried out for 30 min at room temperature and stopped by adding SDS loading buffer and heating at 90 °C for 5 min. Proteins were separated by SDS–PAGE and detected by autoradiography using a Typhoon 9400 imager (GE Healthcare). Two-electrode voltage-clamp recording from Xenopus oocytes The capped RNA (cRNA) was synthesized from 1 μg of linearized plasmid DNA template using an mMessage mMachine in vitro transcription kit (Ambion) according to the manufacturer’s recommendations. The cRNA quality was checked by agarose gel electrophoresis. The concentration was determined by A260/A280 and adjusted to final concentration of 1 μg μl −1 . A total 11.5 ng of each tested cRNA, in a total volume of 46 nl, was injected into each oocyte. Injected oocytes were incubated in ND96 at 18 °C for 2 days prior to electrophysiological. Oocytes were voltage-clamped using a TEV 200 amplifier (Dagan) and monitored by computer through Digidata 1440 A/D converter and pCLAMP 10.2 software (Axon Instruments). The pipette solution contained 3 M KCl. All perfusion buffers contain 48 mM CsCl, 1 mM Ca-gluconate 2 , 1 mM Mg-gluconate 2 , 1 mM K-gluconate, 10 mM Tris/Mes, pH 5.6, unless otherwise noted. Osmolalities were adjusted to 220 mOsmol kg −1 using D -mannitol. During recordings of SLAC1 anion currents, the membrane voltage was stepped to potentials starting at +40 to −140 mV for 7 s with 20-mV decrements and the holding potential was 0 mV. Steady-state currents were extracted at the end of 7-s voltage pulses. For application of intracellular bicarbonate, KHCO 3 was injected into each oocyte. The volume of an oocyte is ~500 nl. The concentrations of free CO 2 and bicarbonate in solutions were calculated using the Henderson–Hasselbalch equation (pH=pK 1 +log[HCO 3 − ]/[CO 2 ]) [57] . Bicarbonate microinjections were performed 20 min before voltage-clamp experiments. How to cite this article: Tian, W. et al . A molecular pathway for CO 2 response in Arabidopsis guard cells. Nat. Commun. 6:6057 doi: 10.1038/ncomms7057 (2015).